Cell-specific alterations inPitx1regulatory landscape activation caused by the loss of a single enhancer 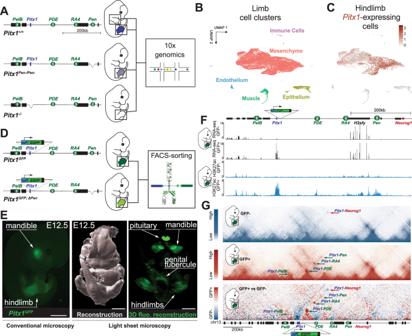Fig. 1: Experimental setup, single cell clustering and regulatory sensor. APitx1+/+,Pitx1Pen−/Pen−, andPitx1−/−transgenic E12.5 embryos were obtained by tetraploid complementation and single cell transcriptomic analyses were produced from fore- and hindlimbs.BUMAP clustering of wildtype and mutant fore- and hindlimbs shows one mesenchymal as well as four satellite clusters.CUMAP colored according toPitx1expression in wildtype hindlimbs (levels represented by the red color scale) shows expression mostly in the mesenchyme cluster.DA cassette containing a minimalβ-globinpromoter (mP) and an EGFP reporter gene is integrated upstream ofPitx1. A secondary round of CRISPR/Cas9 targeting is then used to delete thePenenhancer.EConventional and light-sheet microscopy reveal thatPitx1GFPembryos display EGFP expression domains corresponding to the one ofPitx1(N= 3), scale bars = 2 mm.FRNA-seq and H3K27ac tracks of sorted hindlimb cells show that the sensor approach can separatePitx1active (GFP+) and inactive (GFP−) regulatory landscapes.GC-HiC of thePitx1locus in GFP+ and GFP− hindlimb cells. Darker red or blue bins represent more frequent contacts as represented by scaled bars on the left. GFP+ cells bear chromatin interactions betweenPitx1and its associated enhancers (see green arrows). GFP− cells do not display these interactions but a strong contact betweenPitx1andNeurog1(see red arrow). The lower map is a subtraction of the two above where GFP+ preferential interactions are displayed in red and GFP- preferential interactions in blue. Developmental genes are frequently controlled by multiple enhancers sharing similar specificities. As a result, deletions of such regulatory elements have often failed to reveal their full function. Here, we use the Pitx1 testbed locus to characterize in detail the regulatory and cellular identity alterations following the deletion of one of its enhancers ( Pen ). By combining single cell transcriptomics and an in-embryo cell tracing approach, we observe an increased fraction of Pitx1 non/low-expressing cells and a decreased fraction of Pitx1 high-expressing cells. We find that the over-representation of Pitx1 non/low-expressing cells originates from a failure of the Pitx1 locus to coordinate enhancer activities and 3D chromatin changes. This locus mis -activation induces a localized heterochrony and a concurrent loss of irregular connective tissue, eventually leading to a clubfoot phenotype. This data suggests that, in some cases, redundant enhancers may be used to locally enforce a robust activation of their host regulatory landscapes. Alteration in the enhancer composition of regulatory landscapes at developmental genes can lead to pathologies by modifying the dosage and/or distribution of gene transcription [1] . Indeed, over the past years, losses of single regulatory units within complex and partially redundant regulatory landscapes were shown to have clear phenotypical outcomes despite inducing only partial decreases in average transcription [2] , [3] , [4] , [5] . As the alterations in the regulatory mechanisms following enhancer deletion have mostly been characterized using bulk tissue analysis, it has been difficult to determine the cell-specific variability behind the loss of expression that accounts for phenotypes. In order to understand the precise molecular origin of these phenotypes, it is therefore essential to characterize how a single enhancer contributes to the activation of entire regulatory landscapes in specific cell populations. An effective model system to address these unsolved questions is the limb bud, where organogenesis requires a tight control of gene transcription to achieve correct patterning [6] . Critical to this is Pitx1 , a transcription factor coding gene that is normally expressed in developing hindlimb buds, but not forelimbs, which channels the limb development program to differentiate into a leg [7] , [8] , [9] . Consequently, forelimb Pitx1 gain-of-function can induce an arm-to-leg transformation, featured by the appearance of an ectopic patella as well as complex changes in the muscular and tendons wiring [10] , [11] . In contrast, Pitx1 knock out has been shown to induce partial leg-to-arm transformations with the disappearance of the patella as well as long bone dysplasia and polydactyly [10] , [12] , [13] . Unexpectedly, bulk transcriptomics strategies have only revealed marginal downstream gene expression changes upon Pitx1 loss, suggesting that an interplay between these changes and the growth rate of limb cell subpopulations collectively result in the various phenotypes [8] , [10] , [11] , [13] , [14] . As for many developmental genes, several enhancers coordinate Pitx1 expression in hindlimbs and other tissues. So far, four enhancers have been identified in mammals: PelB which drives a distal reporter pattern in hindlimbs, PDE that drives expression in the mandibular arch, RA4 that can drive reporters in a subset of fore- and hindlimb cells and finally, Pen , a mesenchymal enhancer that drives expression in both fore- and hindlimbs [11] , [15] , [16] . Only the activity of Pen was so far shown to strongly contribute to Pitx1 function in the hindlimb as its deletion leads to a 35–50% reduction of Pitx1 expression [11] . The deletion of Pen has no impact on bone length or digit numbers but induces a partially penetrant clubfoot phenotype, similar to the one observed in mice and humans upon Pitx1 haploinsufficiency [11] , [14] . One particularity to the Pitx1 locus is that it establishes fundamentally different 3D chromatin conformations in transcriptionally active hindlimbs and inactive forelimbs. In active hindlimbs, Pitx1 forms chromatin interactions with cognate cis -regulatory regions spread over 400 kbs, including Pen as well as PDE, RA4 , and PelB . In contrast, in inactive forelimbs these interactions are absent and the Pitx1 gene forms a contact with the polycomb-repressed gene Neurog1 [11] . In this work, we use a combination of single cell transcriptomics (scRNA-seq), a fluorescent cell-tracing approach and genomic technologies to define the contribution of a single enhancer ( Pen ) in establishing the epigenetically- and structurally-active Pitx1 regulatory landscape. Moreover, we investigate whether changes in enhancer activities or 3D structure fundamentally associate with transcription or if those can be functionally disconnected of the transcriptional process. Finally, we assess if Pitx1 expression is homogenous across limb cell populations and if distinct expression levels rely on different enhancer repertoires or, alternatively, in progressive changes in cis-regulatory landscape activities. Two approaches to track Pitx1 activities suggest a bimodal cis -regulatory behavior In order to characterise transcriptional, chromatin and structural changes following the Pen enhancer deletion, we combined genetic manipulation of the Pitx1 locus with scRNA-seq and chromatin analysis of sorted limb cell populations. Both approaches enabled characterization of complementary features of gene transcriptional regulation following alterations of the cis -regulatory landscape. First, to define the hindlimb cell types that are expressing Pitx1 and to assess how the Pen enhancer regulates its expression in these cells, we generated single-cell preparations from wildtype ( Pitx1 +/+ ) fore- and hindlimb buds as well as Pen enhancer deleted ( Pitx1 Pen−/Pen− ) or Pitx1 knocked-out ( Pitx1 −/− ) hindlimbs (Fig. 1A ). We performed 10× genomics in duplicates from E12.5 limb buds as these correspond to a transition stage between patterning and cell-differentiation phases. By performing unsupervised clustering of all the wildtype and mutant single cell transcriptomic datasets, we identified five clusters, to which all the dataset contributed, corresponding to the main populations of the limb: one mesenchymal cluster ( Prrx1 + , Prrx2 + , Twist1 +; 89% of the cells) and four non-mesenchymal satellite clusters including muscle ( Myod1 +, Ttn +; Myh3 +; 4% of the cells), epithelium ( Wnt6 +, Krt14 + ; 5% of the cells), endothelium ( Cdh5 + , Cldn5 +; 1% of the cells) and one immune cell cluster ( C1qa +, Ccr1 +; 1% of the cells) (Fig. 1B , Fig. S1 , Supplementary Dataset S1 ). Yet, as Pitx1 is mostly expressed in the hindlimb mesenchymal cluster, further analyses were performed only in these cells (Fig. 1C ). Fig. 1: Experimental setup, single cell clustering and regulatory sensor. A Pitx1 +/ + , Pitx1 Pen−/Pen− , and Pitx1 −/− transgenic E12.5 embryos were obtained by tetraploid complementation and single cell transcriptomic analyses were produced from fore- and hindlimbs. B UMAP clustering of wildtype and mutant fore- and hindlimbs shows one mesenchymal as well as four satellite clusters. C UMAP colored according to Pitx1 expression in wildtype hindlimbs (levels represented by the red color scale) shows expression mostly in the mesenchyme cluster. D A cassette containing a minimal β-globin promoter ( mP ) and an EGFP reporter gene is integrated upstream of Pitx1 . A secondary round of CRISPR/Cas9 targeting is then used to delete the Pen enhancer. E Conventional and light-sheet microscopy reveal that Pitx1 GFP embryos display EGFP expression domains corresponding to the one of Pitx1 ( N = 3), scale bars = 2 mm. F RNA-seq and H3K27ac tracks of sorted hindlimb cells show that the sensor approach can separate Pitx1 active (GFP+) and inactive (GFP−) regulatory landscapes. G C-HiC of the Pitx1 locus in GFP+ and GFP− hindlimb cells. Darker red or blue bins represent more frequent contacts as represented by scaled bars on the left. GFP+ cells bear chromatin interactions between Pitx1 and its associated enhancers (see green arrows). GFP− cells do not display these interactions but a strong contact between Pitx1 and Neurog1 (see red arrow). The lower map is a subtraction of the two above where GFP+ preferential interactions are displayed in red and GFP- preferential interactions in blue. Full size image In parallel, we devised a fluorescent reporter system to track the regulatory activities of the Pitx1 locus in hindlimbs (Fig. 1D ). Specifically, we first established a reporter line ( Pitx1 GFP ) by homozygously integrating a regulatory sensor cassette, constituted of a minimal β-globin promoter and an EGFP reporter gene, 2 kb upstream of the Pitx1 promoter in mouse embryonic stem cells (mESCs). These cells were re-targeted to obtain a homozygous deletion of the Pen enhancer ( Pitx1 GFP;ΔPen ). 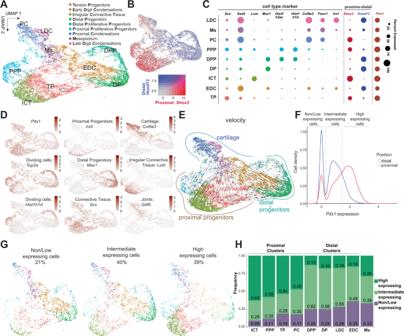Fig. 2:Pitx1expression in wildtype hindlimbs. AUMAP of re-clustered mesenchymal cells from all datasets.BUMAP distribution ofShox2(proximal) andHoxd13(distal) markers. Red to blue heatmap color scale represents levels of expression ofShox2orHoxd13, respectively.CRepresentative marker genes for each cluster. The dot size corresponds to the percentage of cells that express a given marker in the hindlimbPitx1+/+dataset.DUMAP expression distribution of selected marker genes. Red color scales represent selected marker genes levels of expression.ERNA-velocity analysis of hindlimb wildtype mesenchymal clusters. Note that the differentiated chondrocytic cell clusters (upper part) are predicted to derive from proximal and distal progenitors’ clusters (bottom part).FPitx1expression density plot in the proximal (red line) and distal clusters (blue line) in the hindlimb wildtype dataset. Definition of the three types ofPitx1-expressing cells: non/low− (<= 0.3Pitx1expression levels), intermediate- (>0.3; <= 1.45), high- expressing (>1.45). The expression scale corresponds to a logE(expression_value+1).GHindlimb wildtype cells distribution across clusters in the UMAP space based onPitx1expression levels.HHindlimb wildtype cells proportions according toPitx1expression levels across mesenchymal clusters. Embryos were then derived from the mESCs via tetraploid complementation [17] . Conventional and light sheet imaging of Pitx1 GFP embryos showed that the reporter was expressed in all Pitx1 expression domains including the pituitary gland, the mandible, the genital tubercle and the hindlimbs (Figs. 1E , S2A , Supplementary Video S1 ) [13] , [18] , [19] . In order to investigate potential alterations of gene expression following the EGFP transgene integration, we produced E12.5 bulk hindlimb transcriptomes in both Pitx1 +/+ and Pitx1 GFP . Here, we did not observe a change in Pitx1 expression suggesting that the insertion of the EGFP transgene did not alter Pitx1 regulation (Supplementary Dataset S2 ). We then FACS sorted GFP+ and GFP− cells from E12.5 Pitx1 GFP hindlimbs and processed cells for RNA-seq, ChIP-seq and Capture-HiC (C-HiC) (Figs. 1F–G , S2B, C ). We found that 8% of the cells in Pitx1 GFP hindlimbs displayed no EGFP signal, thereby suggesting that the majority of hindlimb cells possesses an active Pitx1 regulatory landscape. We next compared the transcriptome of GFP+ and GFP− cells and observed a 40-fold enrichment for Pitx1 expression in GFP+ cells, validating the Pitx1 GFP allele to track the Pitx1 regulatory landscape activities (Figs. 1F , S3A , Supplementary Dataset S3 ). As expected from our scRNA-seq analyses, we found that GFP+/ Pitx1 + cells were enriched for limb mesenchymal derivatives markers ( Prrx1 , Prrx2, Twist1, Sox9 , Col2a1, Col3a1, Lum ) and that GFP−/ Pitx1 − were enriched for markers of non-mesenchymal satellite clusters including muscle ( Myod1, Ttn ), epithelium ( Wnt6 , Krt15 ), endothelium ( Cdh5 , Cldn5 ) and immune cells ( C1qa , Ccr1 ) (Fig. S3B , Supplementary Dataset S3 ). Yet, the enrichment of these cell types does not preclude a fraction of GFP−/ Pitx1 − to be of mesenchymal origin as we found a weak but clear expression of some mesenchymal markers such as Prrx1 or Twist1 in this population (Fig. S3C ) . Conversely, we found weak expression of muscle ( Myh3 ) and ectodermal ( Krt14 ) markers in GFP +/ Pitx1 + cells (Fig. S3C ). Finally, as Pitx1 was previously associated with tissue outgrowth, we also assayed proliferative and apoptotic behaviors of GFP+ and GFP− cells [20] . As suspected, we found that GFP +/ Pitx1 + cells are slightly more proliferative and contain less apoptotic cells (Fig. S4A, B ). We then assayed the cis -regulatory activities in GFP−/Pitx1− and GFP + /Pitx1 + hindlimb cells using the H3K27ac chromatin mark as a proxy for enhancer activities and C-HiC to determine the locus chromatin architecture [21] . In GFP−/Pitx1− cells, neither Pitx1 promoter nor its various enhancers, including Pen , were found enriched with H3K27ac (Fig. 1F ). Moreover, the locus 3D structure is in a repressed state where Pitx1 displays a strong interaction with the repressed Neurog1 gene and no interaction with its cognate enhancers (Figs. 1G and S5 ). This data shows that GFP−/Pitx1− hindlimb cells display a complete absence of active regulatory landscape features. In contrast, in GFP + /Pitx1 + cells all known Pitx1 enhancers as well as its promoter are strongly enriched in H3K27ac chromatin marks. Furthermore, in these cells Pitx1 establishes strong contacts with its enhancers PelB , PDE, RA4 , and Pen (Figs. 1F, G and S5 ). In summary, this data shows that within the hindlimb, classically considered as a Pitx1 active tissue, 8% of cells, from mesenchymal, immune, endothelium, muscle and epithelium origin, display an inactive Pitx1 cis -regulatory landscape and 3D architecture. Moreover, it suggests a bimodal regulatory behavior, where the Pitx1 promoter, its associated enhancers and the locus 3D structure are all displaying an active mode or none of them are. We then further characterised Pitx1 expression specificities within the hindlimb mesenchyme. Hindlimb proximal cell clusters express Pitx1 at higher level To characterize Pitx1 transcription within mesenchymal subpopulations, we first re-clustered mesenchymal cells from all datasets. From this analysis, we could define nine clusters (Fig. 2A ). We first observed that their distribution in the UMAP space is strongly influenced by the limb proximo-distal axis, as illustrated by Shox2 (proximal marker) and Hoxd13 (distal marker) transcript distributions (Fig. 2B ). We further annotated the clusters according to the expression of known marker genes (Supplementary Dataset S1 ). In the proximal limb section, we identified four clusters. First, we found an undifferentiated P roximal P roliferative P rogenitors cluster which is characterized by high expression of proliferative marker genes, where most cells were found in G2 and S phase and that expresses markers linked to previously identified limb mesenchymal progenitor (LMPs) cells ( PPP : Irx5 +, Alx4 +, Tbx2/3 + , Shox2 + , Hist1h1d +, Top2a +) (Figs. 2C, D and S6A, B ) [22] . We then identified a T endon P rogenitor cluster ( TP : Shox2 +; Osr1 +; Scx +) and an I rregular C onnective T issue cluster which includes muscle connective tissue and ultimately patterns tendons and muscles ( ICT : Shox2 +; Osr1 + , Dcn + , Lum + , Kera + , Col3a1 +) (Fig. 2C, D ) [23] . Finally, in the proximal limb we observed a single cluster of P roximal C ondensations, which already displays late chondrogenic markers and will give rise to proximal limb bones ( PC : Tbx15 +; Sox9 +; Col2a1 +, Col9a3 + , Acan +)(Figs. 2C,D and S6B ) [22] . In the distal limb, we observed the presence of two undifferentiated distal mesenchyme ( Msx1 +) clusters that also relate to previously identified LMPs: one that we classified as D istal P roliferative P rogenitors ( DPP : Tbx2/3 + , Jag1 + , Hoxd13 +; Msx1 +; Hist1h1d +) as it displays a strong expression of proliferation markers, while the other is defined as D istal P rogenitors ( DP : Tbx2/3 + , Jag1 + , Hoxd13 +; Msx1 +) (Figs. 2C, D and S6B ). In both of these clusters a majority of the cells appear to be either in G2 or S phase indicative of their high proliferative rate (Fig. S6A ) . Also, in the distal limb, we identified two more differentiated clusters: E arly D igit C ondensations ( EDC : Hoxd13 + ; Sox9 +, Col2a1− , Col9a3− ), which are a type of distal osteochondrogenic progenitors and L ate D igit C ondensations ( LDC : Irx1 + , Col2a1 + , Col9a3 +) which are more differentiated chondrocytes [22] . Finally, in-between proximal and distal regions ( Shox2 + and Hoxd13 +), we found a cluster of chondrocytic cells that we considered to be the M e s opodium ( Ms : Sox9 +; FoxcI + , Gdf5 + , Col2a1 +) and thus corresponding to ankles or wrists (Fig. 2C, D , Supplementary Dataset S1 ). Fig. 2: Pitx1 expression in wildtype hindlimbs. A UMAP of re-clustered mesenchymal cells from all datasets. B UMAP distribution of Shox2 (proximal) and Hoxd13 (distal) markers. Red to blue heatmap color scale represents levels of expression of Shox2 or Hoxd13 , respectively. C Representative marker genes for each cluster. The dot size corresponds to the percentage of cells that express a given marker in the hindlimb Pitx1 +/+ dataset. D UMAP expression distribution of selected marker genes. Red color scales represent selected marker genes levels of expression. E RNA-velocity analysis of hindlimb wildtype mesenchymal clusters. Note that the differentiated chondrocytic cell clusters (upper part) are predicted to derive from proximal and distal progenitors’ clusters (bottom part). F Pitx1 expression density plot in the proximal (red line) and distal clusters (blue line) in the hindlimb wildtype dataset. Definition of the three types of Pitx1 -expressing cells: non/low− (<= 0.3 Pitx1 expression levels), intermediate- (>0.3; <= 1.45), high- expressing (>1.45). The expression scale corresponds to a logE(expression_value+1). G Hindlimb wildtype cells distribution across clusters in the UMAP space based on Pitx1 expression levels. H Hindlimb wildtype cells proportions according to Pitx1 expression levels across mesenchymal clusters. Full size image To better understand the links between the different clusters, we ran an RNA velocity analysis in the hindlimb dataset, which predicts cell lineage differentiation based on the dynamics of spliced (mature) versus unspliced (immature) mRNAs (Fig. 2E ) [24] , [25] . We found that in the proximal limb a set of Irx5 -expressing cells located within the PPP and ICT clusters are progenitors for the more differentiated proximal clusters such as TP and PC (Fig. 2D, E ) [26] . In the distal limb, DP and DPP clusters appear to be progenitors for EDC and then LDC. The Ms cluster originates from both proximal (PPP-ICT) and distal (DP-DPP) progenitor clusters, confirming its proximo-distal origin (Fig. 2E ). We then assessed whether Pitx1 is differentially expressed among clusters in Pitx1 +/+ hindlimbs. Overall, we found Pitx1 expressed in all mesenchymal clusters, yet with a proximal preference (Fig. 2D, F ). We then classified mesenchymal Pitx1 expressing cells in three categories: non/low-expressing (transcription values < =0.3, 21% of the hindlimb wildtype cells), intermediate-expressing (transcription > 0.3; <= 1.45, 40% of wildtype cells), and high-expressing (transcription > 1.45, 39% of wildtype cells) (Fig. 2F ). As expected, we found that a majority of high expressing cells are located in proximal clusters (PPP, TP, ICT, PC) and a majority of intermediate-expressing cells in distal clusters (DP, DPP, EDC, LDC) (Fig. 2G, H ). We also observed that the Ms cluster, previously identified as a cluster originating from the proximal and distal cell-types, is formed by a similar distribution of high-expressing (proximal) and intermediate-expressing (distal) cells in line with a proximo-distal origin (Fig. 2H ). Pitx1 expression levels associate with global change in regulatory landscape acetylation Next we explored how cells can achieve distinct Pitx1 transcriptional outputs. Practically, we asked whether high- and intermediate-expressing cells use a distinct Pitx1 enhancer repertoire to account for the different expression levels. We sorted the two cell populations from Pitx1 GFP hindlimbs by GFP intensities: GFP+− (intermediate-expressing) and GFP++ (high-expressing) and performed RNA-seq as well as H3K27ac ChIP-seq on the two positive populations (Fig. 3A ). On average, we found three times more Pitx1 transcripts in GFP++ cells than in GFP+− cells as well as an enrichment for several known Pitx1 target genes including Tbx4 (Fig. 3B , Fig. S7A,B , Supplementary Dataset S4 ) [8] . Moreover, as expected from the single-cell analysis, high-expressing GFP++ cells were mostly enriched for proximal limbs markers ( Shox2 , Gsc , Tbx18 , Tbx3 , and Hoxa11 ) and showed higher expression of ICT marker genes ( Kera and Lum ) (Figs. 3C , and S7C , Supplementary Dataset S4 ). In contrast, intermediate-expressing cells GFP+− where enriched for distal cell markers ( Hoxa13 , Hoxd13, Wnt5a , Lhx2 and Msx1 ) (Figs. 3C , S7C , Supplementary Dataset S4 ). Fig. 3: High- and intermediate-expressing Pitx1 regulatory landscape activities. A FACS sorting of Pitx1 GFPs/GFPs forelimb and hindlimbs. Note the EGFP high- (GFP++, dark green) and intermediate-expressing (GFP+−, light green) populations. B . Normalised counts of Pitx1 expression in GFP−, GFP+− and GFP++ cells. Averages are represented by a horizontal bar. Adjusted p -values (padj) of differential gene expression are computed using the Wald-test and Benjamini-Hochberg multiple testing correction as implemented in the Deseq2 tool (Supplementary Dataset S4 and Source data). C Expression of selected marker genes in GFP− (satellite cell types), GFP+− (distal) and GFP++ (proximal and ICT) cells. D H3K27ac ChIP-seq at the Pitx1 locus. Note that enhancers are active in both intermediate- and high-expressing cells, yet with a few regions marked only in high-expressing cells. E H3K27ac profile at the Pitx1 gene body, Pitx1 Proximal Promoter Region (PPPR, see black arrow), region A (regA), PDE and Pen enhancer. Full size image In both intermediate- and high-expressing cells, the previously characterized Pitx1 enhancer repertoire— PelB , PDE , RA4 , and Pen —was found marked by H3K27ac. Yet, in high-expressing cells (GFP++), stronger H3K27ac signal was found at these elements concomitantly with a strong increase at two specific regions: the Pitx1 proximal promoter region ( PPPR ) and the region A ( regA ). We also observed a few regions upstream of Pen that were strongly enriched for H3K27ac in GFP++ cells (Fig. 3D, E ) [11] . However, those sequences do not seem to be important for Pitx1 expression as the deletion of the entire region between Pitx1 and Pen , including Pen but not those regions, fully recapitulates the Pitx1 hindlimb knock out phenotype [11] . Altogether, this data shows that Pitx1 regional expression differences across hindlimbs associate with a progressive increase of its cis -regulatory landscape activity rather than from the usage of different enhancers repertoires. These results further re-enforce the idea that the fundamental unit of Pitx1 regulation is the landscape as a whole rather than individual enhancers. Pen deletion increases the proportion of Pitx1 non/low-expressing cells in hindlimbs Observing the coordination between regulatory units at the locus to modulate gene expression, we sought to test how the deletion of one of them influences the overall unity of the locus. Therefore, we took advantage of the Pitx1 EGFP sensor and of scRNA-seq to track how the homozygous deletion of the Pen enhancer affects the hindlimb Pitx1 locus activity. First, the removal of Pen within the Pitx1 GFP background ( Pitx1 GFP;ΔPen ) induced a shift in the expression of the GFP reporter gene in hindlimbs (Fig. 4A, B ). Specifically, the proportion of GFP− cells raised from 8% in Pitx1 GFP to 16% in Pitx1 GFP;ΔPen at E12.5 and from 12% to 29% at E13.5 (Fig. S8A, B ). To confirm that this effect is not due to a difference in the distribution of EGFP fluorescence during cell sorting, we compared EGFP transcription in Pitx1 GFP;ΔPen and Pitx1 GFP GFP− cells and did not observe a difference (Fig. S8C ). Fig. 4: Influence of the Pen deletion on Pitx1 expression in hindlimb cell populations. A EGFP expression pattern in Pitx1 GFP and Pitx1 GFP;ΔPen E12.5 embryos ( N = 3), scale bar = 2 mm. B FACS profile of Pitx1 GFP (red) and Pitx1 GFP;ΔPen (cyan) hindlimbs shows an increased number of EGFP non/low-expressing cells as well as a decrease of EGFP high-expressing cells in Pitx1 GFP;ΔPen hindlimbs. C Pitx1 expression distributions in Pitx1 +/+ (red) and Pitx1 Pen−/Pen− (cyan) hindlimb cells show an increased proportion of non/low-expressing cells and a decreased proportion of high-expressing cells in Pitx1 Pen−/Pen− hindlimbs. The dotted lines indicate the threshold between non/low-expressing and intermediate-expressing (0.3) as well as between intermediate-expressing and high expressing cells (1.45). The expression scale is a logE(expression_value+1). D Pitx1 expression across all clusters in Pitx1 +/+ and Pitx1 Pen−/Pen− hindlimbs. Averages are represented by a horizontal bar. Adjusted p -values ( p ) shown in the figure were calculated by Wilcoxon Ranks Sum test using the FindMarkers function from Seurat R Package (Supplementary Dataset S5 ). The dotted lines indicate the threshold between non/low-expressing and intermediate-expressing (0.3). The fold change in non/low-expressing cell number between Pitx1 +/+ and Pitx1 Pen−/Pen− is shown at the bottom of the violin plots. Note the strong loss of expression and the accumulation of non/low-expressing cells in ICT and PPP clusters. E Distribution of Pitx1 expression in proximal and distal cells of Pitx1 +/+ and Pitx1 Pen−/Pen− hindlimbs. Note the strong increase in proximal non/low-expressing cell fraction. F Proportion of non/low-, intermediate- and high- Pitx1 expressing cells across conditions. Full size image Secondly, we compared Pitx1 +/+ and Pitx1 Pen−/Pen− scRNA-seq dataset and found a similar effect as the Pen deletion induces a significant 29% loss of Pitx1 expression (adjusted p -value = 1.75e−96 (Wilcoxon Rank Sum test)) featured by a decrease in Pitx1 high-expressing cells and a strong increase in non/low-expressing cells (Fig. 4C ). Across hindlimb mesenchymal cells, the proportion of non/low-expressing cells was indeed raised from 21% in Pitx1 +/+ to 35% in Pitx1 Pen−/Pen− . In summary, the two approaches show that behind the weak average loss of Pitx1 expression, a strong increase of non/low-expressing cells in mutant hindlimbs could account for the clubfoot phenotype seen in these animals [11] . We further quantified within the scRNA-seq dataset if this alteration in expression was equally distributed among various hindlimb cell-types or if some populations were more specifically affected. All clusters with the exception of the Ms and the LDC showed a significant loss of Pitx1 expression ranging from 24 to 39% (Fig. 4D ). With respect to the proportion of non/low-expressing cells, we saw that proximal cells showed a preferential 2.1-fold enrichment of non/low-expressing cells (13 to 28%) in comparison with distal cells (1.6-fold, 29 to 45%) (Fig. 4E, F ). We then computed the increase of non/low-expressing Pitx1 cells in each cluster and saw that two proximal clusters, ICT and PPP, showed a particularly strong 3.5- and 2-fold increase in Pitx1 non/low-expressing cells respectively (Fig. 4D ). It is important to note that in both clusters the vast majority of cells usually express Pitx1 at a high level (Figs. 2H , S9 ). Other clusters showed 1.5- to 1.8-fold increase in Pitx1 non/low-expressing cells. In conclusion, we found that proximal, high-expressing clusters are more affected by the enhancer deletion than distal, intermediate-expressing clusters. We subsequently investigated if this differential alteration of Pitx1 expression among hindlimb cell population affected the proportion of cells within the clusters. Pen deletion delays the formation of irregular connective tissue As a positive control for the effect of Pitx1 loss-of-function in Pitx1 Pen−/Pen− embryos, we took advantage of two datasets that do not express Pitx1 : Pitx1 +/+ forelimbs and Pitx1 −/− hindlimbs. As a proxy for the functional impact of Pitx1 transcriptional change on limb development, we measured the relative proportions of the different cell clusters in the different datasets. First, we did not observe changes in the proportions of non-mesenchymal satellite cell clusters in any of the conditions (Fig. S10 ). We then measured the proportions of the different mesenchymal sub-clusters (Fig. 5A, B ). By comparing wildtype fore- and hindlimbs, we did not observe any significant change in the proportion of cell-types, suggesting that fore- and hindlimbs are similarly populated despite the obvious structural differences between arms and legs. In contrast, Pitx1 −/− hindlimbs display a heterochronic phenotype, featuring an increase in progenitor cells in both the proximal and distal regions of hindlimbs (PPP and DPP cell clusters) while a concurrent decrease is seen in several differentiated cell types in proximal and distal hindlimbs (ICT, PC, Ms, and LDC) (Fig. 5A, B ). Remarkably, the loss of the Pen enhancer resulted in a similar effect but only significant in the proximal limb cell clusters (Fig. 5A, B ). Specifically, the proportion of PPP cells increased in Pitx1 Pen−/Pen− hindlimbs as the proportion of ICT cells decreased. This alteration correlates with the strong loss of Pitx1 transcription seen in both clusters (Fig. 4D ). The increase in PPP cells is further supported by the upregulation of its markers in Pitx1 Pen−/Pen− hindlimbs ( Hist1h genes, Top2a , and others; Supplementary Dataset S5 ). Fig. 5: Influence of the Pen deletion on limb cell populations. A UMAP of mesenchymal cell type proportions across conditions, (+) and (−) symbols indicate increase or decrease in cell proportions in comparison to wildtype hindlimbs. Abbreviations are described in Fig. 2A . B Quantification of cell type proportions across conditions, p -values < 0.01 are marked with an asterisk (see Source data). P -values were calculated pairwise using differential proportion analysis in R [60] . Abbreviations are described in Fig. 2A . C Velocity analyses from proximal clusters in all dataset. Arrows represent the direction toward the predicted fate territories. Note in Pitx1 Pen−/Pen− and Pitx1 −/− the velocity-predicted cell movements between PPP and ICT which likely represent ongoing differentiation that is not predicted in wildtype hindlimbs or forelimbs. D Velocity analyses from distal clusters in all dataset. Note in Pitx1 −/− hindlimbs the loss of late digit condensations (black arrows) at the end of the velocity-predicted cell movements. Full size image To test if these effects could be explained by a delayed differentiation of progenitor cells, we performed a velocity analysis on Pitx1 −/− , Pitx1 Pen−/Pen− and Pitx1 +/+ limbs in proximal and distal cell clusters separately. In the proximal part of the hindlimb, we found in both mutants a predicted connection from PPP to ICT cells, suggesting an ongoing differentiation process (Fig. 5C ). This connection was not present in Pitx1 +/+ fore- and hindlimbs, suggesting that the differentiation process was completed in these tissues. These findings are further supported by an increase of ICT marker genes ( Lum , Dcn , and Kera ) in PPP cells of both mutants, suggesting that those cells have only partially adopted an ICT identity but still did not fully differentiate (Fig. S11 ). In contrast, the velocity analysis of distal clusters did not show any changes in Pitx1 Pen−/Pen− hindlimbs, in agreement with the unaltered proportion of distal cell clusters shown above (Fig. 5B, D ). Finally, we observed in Pitx1 −/− hindlimbs an accumulation of distal progenitor cells and a loss of differentiated LDC cells suggesting a slower distal differentiation process in Pitx1 −/− hindlimbs. Together, these findings support a form of heterochrony that affects only the proximal part of Pitx1 Pen−/Pen− hindlimbs and that is featured by a delayed differentiation of PPP to ICT. As Pitx1 has been shown to have both indirect and direct downstream effects, we further investigated differentially expressed genes in Pitx1 loss-of-function hindlimbs that could induce these effects. In particular it has been shown that Tbx4 , a known downstream target gene of Pitx1 , mediates the Pitx1 -effect on hindlimb buds growth rate [8] , [20] , [27] . 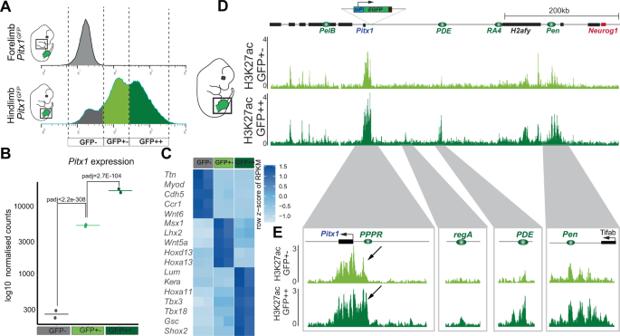Fig. 3: High- and intermediate-expressingPitx1regulatory landscape activities. AFACS sorting ofPitx1GFPs/GFPsforelimb and hindlimbs. Note the EGFP high- (GFP++, dark green) and intermediate-expressing (GFP+−, light green) populations.B. Normalised counts ofPitx1expression in GFP−, GFP+− and GFP++ cells. Averages are represented by a horizontal bar. Adjustedp-values (padj) of differential gene expression are computed using the Wald-test and Benjamini-Hochberg multiple testing correction as implemented in the Deseq2 tool (Supplementary Dataset S4 and Source data).CExpression of selected marker genes in GFP− (satellite cell types), GFP+− (distal) and GFP++ (proximal and ICT) cells.DH3K27ac ChIP-seq at thePitx1locus. Note that enhancers are active in both intermediate- and high-expressing cells, yet with a few regions marked only in high-expressing cells.EH3K27ac profile at thePitx1gene body,Pitx1Proximal Promoter Region (PPPR, see black arrow), region A (regA),PDEandPenenhancer. As anticipated, we found a downregulation of the Tbx4 in all clusters aside of PC, Ms, and LDC in both Pitx1 −/− and Pitx1 Pen−/Pen− hindlimbs, with the strongest effect in ICT and PPP clusters (Fig. S12A–D , Supplementary Dataset S5 ). To further determine the origin of the Tbx4 loss we assessed in Pitx1 Pen−/Pen− hindlimb clusters the expression of caudal Hox genes, which have been suggested to control Tbx4 along with Pitx1 [28] . Here, we did not find an alteration in Hox expression levels that correlates with Tbx4 loss, suggesting that Tbx4 decrease is rather a direct effect of Pitx1 loss-of-expression (Supplementary Dataset S5 ). Finally, we measured if the Tbx4 expression loss was sufficient to alter cell proliferation and apoptosis, therefore changing the hindlimb cell type composition [20] . Overall, we did not observe changes in either, suggesting that the observed loss of Tbx4 is not sufficient to alter cell proliferation and apoptosis, and that the induced phenotype takes origin from an independent mechanism (Fig. S13A, B ). Moreover, aside from Tbx4 , we found numerous dysregulated genes in Pitx1 Pen−/Pen− hindlimbs which might contribute to observed phenotypes (Supplementary Dataset S5 ). This is the case for Dcn , an ICT marker gene previously described to be involved in tendon elasticity in mice as well as the Six1 and Six2 genes that are expressed in connective tissue and necessary for skeletal muscle development [23] , [29] , [30] , [31] , [32] . The Pen enhancer contributes to Pitx1 regulatory landscape activation The establishment of the active Pitx1 chromatin landscape includes changes in 3D conformation and the acetylation of specific cis -regulatory elements. Therefore, we asked whether the Pen enhancer itself is required to establish these features and specifically if its deletion would impact them. In GFP+ and GFP− cells from Pitx1 GFP;ΔPen hindlimb buds, we used RNA-seq to assess whether we could observe similar changes in cellular identity upon Pen enhancer loss as the one previously described using scRNA-seq. As expected, we could observe in GFP− cells the accumulation of mesenchymal markers ( Prrx1 , Twist1 ) with a particular enrichment for ICT markers ( Col3a1, Col1a1, Col1a2, Lum) (Fig. 6A , Supplementary Dataset S6 ). As a consequence of the accumulation of Pitx1 non/low-expressing mesenchymal cells, we also observed a dilution of non-mesenchymal clusters marked by a decrease of epithelium ( Wnt6 , Krt14 ) and muscle ( Ttn ) markers. In GFP+ cells, we did not observe a clear change in identity markers indicating that the cell type composition is similar between Pitx1 GFP and Pitx1 GFP;ΔPen high-expressing cells (Supplementary Dataset S7 ). This suggests that these high expressing cells, that escape a loss-of-expression following the deletion of Pen , must display an adaptive mechanism to accommodate the Pen enhancer loss. Fig. 6: Single enhancer deletion results in inefficient regulatory landscape activation. A Log2 fold change and RPKM of mesenchymal (red) and satellite (darkgreen) marker genes in Pitx1 GFP and Pitx1 GFP;ΔPen GFP− hindlimbs cells. Note the decrease in satellite markers and the increase in mesenchymal markers in Pitx1 GFP;ΔPen GFP− cells. B H3K27ac ChIP-seq and RNA-seq tracks at the Pitx1 locus in GFP+ cells of Pitx1 GFP and Pitx1 GFP;ΔPen hindlimbs. Note the loss of the Pen enhancer region (black arrow). C H3K27ac ChIP-seq and RNA-seq at the Pitx1 locus in GFP− cells of Pitx1 GFP and Pitx1 GFP;ΔPen hindlimbs. Note the acetylation of Pitx1 promoter and enhancers (blue arrows) and the weak Pitx1 transcription. D C-HiC subtraction map between GFP− and GFP+ Pitx1 GFP;ΔPen hindlimb cells. GFP+ preferential interactions are displayed in red and GFP- preferential interactions in blue. E C-HiC subtraction maps between Pitx1 GFP and Pitx1 GFP;ΔPen GFP+ hindlimb cells. Note the loss of interaction between Pitx1 and the Pen- deleted region (green arrow). Pitx1 GFP;ΔPen GFP+ preferential interactions are displayed in red and Pitx1 GFP GFP+ preferential interactions in blue. F Subtraction track of virtual 4C between Pitx1 GFP (blue) and Pitx1 GFP;ΔPen (red) GFP+ hindlimb cells with the Pitx1 promoter as viewpoint. Note the partial loss of interactions between Pitx1 and its telomeric enhancers ( PDE, RA4 , and Pen ; green arrows). G C-HiC subtraction maps between Pitx1 GFP and Pitx1 GFP;ΔPen GFP− hindlimb cells. Pitx1 GFP;ΔPen GFP− preferential interactions are displayed in red and Pitx1 GFP GFP− preferential interactions in blue. Full size image We then performed H3K27ac ChIP-seq in the escaping GFP+ cells and in the increased fraction of GFP− cells. In Pitx1 GFP;ΔPen GFP+ cells, we observed a distribution of H3K27ac over the landscape that was virtually identical to Pitx1 GFP GFP+ hindlimbs cells, with the exception of the Pen enhancer itself (Fig. 6B ). This result suggests that the Pitx1 expressing cells in the Pen deletion background use the same enhancer repertoire as the Pitx1 GFP expressing cells and thus do not use an alternative regulatory landscape. Moreover, we observed the same average Pitx1 expression level in Pitx1 GFP and Pitx1 GFP;ΔPen GFP+ cells (Supplementary Dataset S7 ). In GFP− cells deleted for Pen , in contrast to Pitx1 GFP cells, we observed ectopic acetylation of the Pitx1 promoter as well as of the RA4 and PelB enhancers (Fig. 6C ). These activities are likely caused by the relocation, in the GFP− fraction, of cells that would normally express Pitx1 but fail to establish a fully active landscape in the absence of Pen . In these cells, we observed a marginal increase in Pitx1 expression (FC = 1.6, padj = 0.0026) that suggests that the locus is less repressed as in wildtype GFP− cells (Fig. 6C , Supplementary Dataset S6 ). We then measured how the lack of Pen affects the locus 3D structure dynamics in Pitx1 GFP;ΔPen hindlimbs. 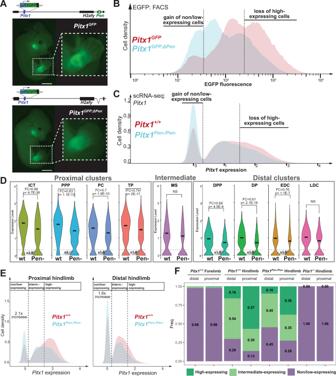Fig. 4: Influence of thePendeletion onPitx1expression in hindlimb cell populations. AEGFP expression pattern inPitx1GFPandPitx1GFP;ΔPenE12.5 embryos (N= 3), scale bar = 2 mm.BFACS profile ofPitx1GFP(red) andPitx1GFP;ΔPen(cyan) hindlimbs shows an increased number of EGFP non/low-expressing cells as well as a decrease of EGFP high-expressing cells inPitx1GFP;ΔPenhindlimbs.CPitx1expression distributions inPitx1+/+(red) andPitx1Pen−/Pen−(cyan) hindlimb cells show an increased proportion of non/low-expressing cells and a decreased proportion of high-expressing cells inPitx1Pen−/Pen−hindlimbs. The dotted lines indicate the threshold between non/low-expressing and intermediate-expressing (0.3) as well as between intermediate-expressing and high expressing cells (1.45). The expression scale is a logE(expression_value+1).DPitx1expression across all clusters inPitx1+/+andPitx1Pen−/Pen−hindlimbs. Averages are represented by a horizontal bar. Adjustedp-values (p) shown in the figure were calculated by Wilcoxon Ranks Sum test using the FindMarkers function from Seurat R Package (Supplementary DatasetS5). The dotted lines indicate the threshold between non/low-expressing and intermediate-expressing (0.3). The fold change in non/low-expressing cell number betweenPitx1+/+andPitx1Pen−/Pen−is shown at the bottom of the violin plots. Note the strong loss of expression and the accumulation of non/low-expressing cells in ICT and PPP clusters.EDistribution ofPitx1expression in proximal and distal cells ofPitx1+/+andPitx1Pen−/Pen−hindlimbs. Note the strong increase in proximal non/low-expressing cell fraction.FProportion of non/low-, intermediate- and high-Pitx1expressing cells across conditions. First, GFP+ and GFP− Pitx1 GFP;ΔPen hindlimb cells displayed differences similar to their Pitx1 GFP active and inactive counterparts (Figs. 1F , 6D , S14A ). This suggests that escaping high-expressing hindlimb Pitx1 GFP;ΔPen cells do not require Pen to establish an active 3D conformation. We then asked whether these cells bare an alternative chromatin structure than wildtype ones to compensate for the loss of Pen . By comparing Pitx1 GFP and Pitx1 GFP;ΔPen GFP+ cells we saw no major differences (Figs. 6E , S14B ). Yet, using virtual 4C, we saw a slight reduction of contacts between the Pitx1 promoter and PDE/RA4 in GFP+ cells (Figs. 6F , S14D ). This suggests that the remaining high-expressing cells do not necessarily undergo a strong adaptive structural response to the loss of Pen to ensure high Pitx1 expression. Finally, we asked whether the relocated Pitx1 GFP;ΔPen GFP− cells, that bear ectopic promoter and enhancer acetylation, display features of an active 3D structure (Figs. 6G , S14C, D ). However, we did not observe any changes in the Pitx1 locus conformation in these cells in comparison to Pitx1 GFP GFP− cells. This shows that despite some remaining regulatory activity (evidenced by low level H3K27ac; arrows Fig. 6C ), the locus is unable to assume its active 3D structure and therefore to efficiently transcribe Pitx1 (Fig. 6G ). In conclusion, the Pen enhancer is necessary to ensure that all the cells with active enhancers at the Pitx1 locus undergo a robust transition toward a structurally and transcriptionally active landscape (Fig. 7 ). Fig. 7: Model. In wildtype hindlimb tissues (left panel) 8% of the nuclei, mostly from non-mesenchymal origin, display a completely repressed Pitx1 locus, featured by inactive enhancers (white ovals), polycomb-repressed Pitx1 gene (red rectangle) and inactive 3D chromatin structure ( Pitx1 does not contact its enhancers but contacts the repressed Neurog1 gene). In active nuclei, the situation is inverted with active enhancers (green ovals), active 3D chromatin structure ( Pitx1 contacts its enhancers) and strong Pitx1 transcription. In contrast, in hindlimb lacking the Pen enhancer (right panel), 16% of the cells are lacking Pitx1 transcription. Among these cells, some display a partially active regulatory landscape. These latter cells, that have failed to establish an active 3D structure and a strong Pitx1 transcription, are of mesenchymal origins in particular of ICT and PPP types. The remaining active cells in mutant hindlimbs appear to display wildtype expression levels. Phenotypically, the effect of the enhancer deletion is a disharmonious outgrowth of cell populations featured by a gain of PPP and a decrease of ICT cells. This cellular phenotype is likely at the origin of the clubfoot phenotype. Full size image In this work we have shown that hindlimb cells display several states of Pitx1 regulatory activities. In active cells, all enhancers are marked with the active H3K27ac chromatin modification and are contacting the Pitx1 promoter. In contrast, in inactive cells, we could not observe partial regulatory activities, i.e. neither enhancer acetylation nor enhancer-promoter interactions. This shows that the locus follows a bimodal behavior where the regulatory landscape as a whole acts on Pitx1 transcription. Indeed, a common set of coordinated enhancers are active in both proximal Pitx1 high-expressing and distal Pitx1 low-expressing cells. In fact, the Pitx1 regulatory landscape acts here similarly to what was previously defined as a holo-enhancer, where the whole region seems to work as a coherent regulatory ensemble [33] . In this perspective, Pitx1 expression levels are adjusted by the entire landscape. This is what we observed in high Pitx1 -expressing proximal cells where the same enhancer set than in distal cells displays a higher enrichment for the active H3K27ac chromatin mark along with a few proximal-specific regions that are more enriched for H3K27ac. This suggests that proximal transcription factors or signaling cues are controlling the landscape either by binding simultaneously at several Pitx1 cis -regulatory regions or by targetedly modifying other parameters of locus activity such as the frequencies of active chromatin interactions or the proximity to the repressive nuclear lamina for instance. Here we have tested how the loss of one of the regulatory elements, the Pen enhancer, which is conserved among all tetrapods and required for hindlimb identity, affects the establishment of the Pitx1 active landscape [11] , [34] . Some escaping cells can induce Pitx1 regulatory landscape activation without Pen , suggesting that the other cis -regulatory modules ( PelB , PDE , and RA4 ) provide a form a compensation. These modules are likely activated by a similar gene-regulatory network in wildtype and mutant hindlimbs, as we could not observe a clear shift in cell identity of GFP/Pitx1 expressing cells. Alternatively, a cumulative effect of marginal transcriptional changes in cell identity along with specific non-transcriptional identity differences could maintain the capacity of cells to generate a high Pitx1 expression level despite the absence of Pen . Simultaneously, many Pitx1 low/non-expressing cells accumulate in hindlimbs that bear enrichment of H3K27ac at the Pitx1 promoter and at several of its enhancers (Fig. 7 ). Despite the presence of this active modification, the Pitx1 locus does not adopt an active 3D chromatin folding but maintains the hallmarks of its inactive configuration. In fact, these accumulated low/non-expressing cells are seemingly stuck in a limbo between activity and repression and show the importance of the coordinated action of enhancer activity and 3D chromatin changes to achieve sufficient transcriptional strength. Therefore, we hypothesize that the role of Pen is not to act as a pattern-defining enhancer but rather as a support enhancer that ensures a robust transition of cells towards a fully active Pitx1 landscape and therefore a strong Pitx1 transcription. Here, other enhancers, such as RA4 , PelB as well as other to be defined enhancers, might bear this pattern-defining role. In fact, Pen is a good model to understand the fundamental role of many enhancers that were characterised with a diverging activity than the gene they control [35] , [36] , [37] . This “class” of enhancers would therefore govern the cooperativity of loci’s regulatory landscapes without defining by themselves their expression specificities. Changes in the number of cells that express Pitx1 in the hindlimb have strong phenotypical consequences. In fact, the complete loss of Pitx1 induces an increase in proximal and distal progenitor cells concomitantly with a loss of differentiated cell types, overall altering the proportion of specific cell clusters in hindlimbs. The global increase in progenitors indicates a heterochrony in limb development that ultimately results in a reduction of the limb size and the loss of some limb structures such as the patella. In the case of the Pen enhancer deletion, we saw an enrichment of Pitx1 low/non-expressing cells in PPP and ICT clusters resulting in a delayed differentiation of PPP into ICT. Although the reduction of Pitx1 transcription induces the decrease of its direct target, Tbx4 , involved in limb bud outgrowth and cell proliferation, it was here not sufficient to alter cell proliferation or apoptotic rates, at E12.5, suggesting that the clubfoot phenotype builds on a Tbx4 -independent differentiation problem [20] , [27] . Here, the particularly strong effect of the Pen deletion on the ICT cell proportion pinpoints these cells as the origin of the clubfoot phenotype seen in mice lacking the enhancer. In fact, ICT has been repeatedly reported to function in a non-cell autonomous way during limb development and to act as an important driver of muscle patterning [23] , [38] , [39] , [40] , [41] , [42] , [43] . We, therefore, suspect that the loss of ICT in hindlimbs leads to a muscle patterning defect which would be at the base of the clubfoot phenotype. Moreover, the observed heterochrony in several of the mesenchymal cell populations could collectively cause the clubfoot since coordinated expansion and interactions among different mesenchymal cell populations are required for normal limb morphogenesis. Finally, despite lacking Pitx1 expression as well, forelimb cell clusters are present in the same proportion as hindlimb ones. This suggests that the role of Pitx1 in hindlimbs is mirrored by other genes in forelimbs, such as Tbx5 , that account for a harmonious outgrowth of the various cell populations. Indeed, Tbx5 loss of expression in the ICT population alters muscle and tendons patterning causing the mice to hold the paw in a supine position, leading them to walk on the edge or dorsal surface of the paw, resembling a clubfoot phenotype [23] . Our characterization of a single enhancer loss-of-function mutant at a cell subpopulation level opens the way to study the effect of other regulatory mutations with the same resolution and, in particular, of gain-of-function mutations. Such approaches will enable to select particular cell-subpopulations that show ectopic transcription in comparison to neighboring cells that bear the same mutation but no ectopic expression. This will facilitate a precise definition of features that are permissive for transcriptional gain-of-function and will be an important tool to further investigate the relationship between 3D structure, chromatin modifications, and gene transcriptional activation. Cell culture, mice and tissue processing Animal procedures All animal procedures were in accordance with institutional, state, and government regulations (Canton de Genève authorisation: GE/89/19). CRISPR/Cas9 engineered alleles Genetically engineered alleles were generated using the CRISPR/Cas9 editing according to ref. [44] . Briefly, sgRNAs were designed using the online software Benchling and were chosen based on predicted off-target and on-target scores. All sgRNAs and target genomic locations for CRISPR–Cas9 can be found in Supplementary Table S1 . SgRNAs were then sub-cloned in the pX459 plasmid from Addgene and 8 μg of each vector was used for mESCs transfection. mESCs culture and genetic editing followed standard procedure [45] . To construct the Pitx1 GFP mESCs clone, the LacZ sensor from [11] was adapted by exchanging the LacZ by an EGFP cassette. The sgRNA was designed to target CRISPR–Cas9 to chr13:55935371-55935390 (Supplementary Table S1 ). Cells were transfected with 4 μg of EGFP−cassette and 8 μg of pX459 vector containing the sgRNA. Transgenic G4 ESCs clones can be obtained upon request. Aggregation of mESC Embryos were generated by tetraploid complementation from G4 male ESCs obtained from the Nagy laboratory ( http://research.lunenfeld.ca/nagy/?page=mouse%20ES%20cells ) [17] , [46] . Desired mESCs were thawed, seeded on male and female CD1 feeders and grown for 2 days before the aggregation procedure. Donor tetraploid embryos were provided from in vitro fertilisation using c57bl6J x B6D2F1 backgrounds. Aggregated embryos were transferred into CD1 foster females. All animals were obtained from Janvier laboratories. Single-cell RNA-seq dissociation Two replicates of fore and hindlimb buds of E12.5 wildtype embryos and hindlimb buds of mutant embryos ( Pitx1 Pen−/Pen− , Pitx1 −/− ) were micro-dissected and incubated for 12 min in 400 μl trypsin-EDTA 0.25% (Thermo Fischer Scientific, 25300062), supplemented with 40 μl of 5% BSA. During incubation tissues were disrupted by pipetting after 6 min of incubation and at the end of the 12 min. Trypsin was then inactivated by adding 2× volume of 5% BSA and single cell suspension was obtained by passing cells in a 40 μm cell strainer. Cells were then spun at 250 × g for 5 min at 4 °C and resuspended in 1%BSA in PBS. Cells were then counted using an automatized cell counter and a 1% BSA 700 cells/μl suspension was prepared. 10 μl of this solution was used as input for the 10× Genomics library preparation. Single-cell library preparation Single-cell libraries were prepared using the Chromium Single Cell 3′ GEM, Library & Gel Bead Kit v3 following the manufacture’s protocol (10× Genomics, PN-1000075). Briefly, Gel beads in EMulsion (GEMs) are generated by combining Single Cell 3′ v3 Gel Beads, a Master Mix containing cells, and Partitioning Oil onto Chromium Chip B. Incubation of the GEMs produced from the poly-adenylated mRNA barcoded, full-length cDNA. Immediately, gel beads are dissolved and cDNA is amplified via PCR followed by library construction and sequencing. Libraries were paired-end sequenced on a HiSeq 4000. On average, 7000 cells were loaded on the Chromium Chip and between 25,000 and 35,000 mean reads were obtained. Whole-mount in situ hybridization (WISH) Pitx1 WISH were performed on 40–45 somite stage mouse embryos (E12.5) using a digoxigenin-labeled Pitx1 antisense riboprobe transcribed from a cloned Pitx1 probe (PCR DIG Probe Synthesis Kit, Roche), as previously described in ref. [11] . Light sheet microscopy imaging E12 embryos post-fixed overnight in 4% PFA. Tissue was cleared using passive CLARITY based clearing method. Briefly, tissue was incubated in a Bis-free Hydrogel X-CLARITY™ Hydrogel Solution Kit (C1310X, Logos Biosystems) for 3 days at 4 °C, allowing diffusion of the hydrogel solution into the tissue. Polymerization of solution was carried in a Logos Polymerization (C20001, Logos Biosystem) system at 37 °C for 3 h. (SDS-Clearing solution: For 2 L of 4% SDS solution used 24.73 g of boric acid (Sigma B7660 or Thermofisher B3750), 80 g of sodium dodecyl sulfate (Brunschwig 45900-0010, Acros 419530010 or Sigma L3771), in dH 2 O, final solution pH 8.5). After two washes of 30 min in PBS, samples were immersed in a SDS based clearing solution and left at 37 °C for 48 h. Once cleared, tissue was washed twice in PBS-TritonX 0.1% and then placed in a Histodenz© based-refractive index-matching solution (Histodenz Sigma D22158, PB + Tween + NaN 3 pH 7.5 solution, 0.1% Tween-20, 0.01% NaN 3 , in 0.02 M phosphate buffer, final solution pH 7.5) Imaging was performed with a home-built mesoscale single-plane illumination microscope; complete description of the mesoSPIM microscope is available here: (Voigt et al. [47] ). Briefly, using one of the two excitation paths, the sample was excited with 488 and 561 nm laser. The beam waist was scanned using electrically tunable lenses (ETL, Optotune EL-16-40-5D-TC-L) synchronized with the rolling shutter of the sCMOS camera. This produced a uniform axial resolution across the field-of-vie7w (FOV) of 5 μm. GFP autofluorescence signal was filtered with 530/43 nm, 593/40 nm bandpass filter (BrightLine HC, AHF). Z-stacks were acquired at 5 μm spacing with a zoom set at ×1.25 resulting in an in-plane pixel size of 5.26 μm. Images were pre-processed to subtract the background and autofluorescence signal using the 561 nm excitation channel and subsequent normalization and filtering of the images were performed with the Amira 2019.4 software. 3D videos and images were captured using the Imaris 9.5 software. Tissue collection and cell preparation for FACS-sorting Forelimb and hindlimb buds from embryos with 40–45 somites (E12.5) were dissected in cold PBS solution. After PBS removal, a single cell suspension was achieved by incubating the limb buds in 400uL Trypsin-EDTA (Thermo Fischer Scientific, 25300062) for 12′ at 37 °C in a Thermomixer with a resuspension step at the 6′ mark. After blocking with one volume of 5% BSA (Sigma Aldrich, A7906-100G), cells were passed through a 40 μm cell strainer for further tissue disruption and another volume of 5% BSA was added to the cell strainer to pass leftover cells. Cells were then centrifuged at 400 × g for 5′ at 4 °C and, after discarding the supernatant, they were resuspended in 1% BSA for cell sorting. 5 mM of NaButyrate were added to the BSA when planning for subsequent fixation for H3K27Ac-ChIP. Proliferation and apoptosis analyses After tissue collection and cell dissociation, apoptotic cells were identified through Annexin V staining (Invitrogen, R37177). Following the manufacturer’s instructions, two replicates of 2 × 10 5 cells were resuspended in the kit’s binding buffer and 1 drop of Annexin V stain was added per 1 × 10 5 cells and left at room temperature incubation for 15′. Apoptotic phases were then determined by flow cytometry analysis. For cell cycle analysis we used two replicates of 2 × 10 5 cells, where DNA was stained with Hoechst-33342 dye (Abcam, ab228551) used to a final concentration of 5 μg/ml in a 1% BSA media. Cells were left for a 30′ incubation in a 37 °C water bath. Flow cytometry was then used to determine cell cycle stage. Both experiments were performed on a BDLSR Fortessa analyser and data was then processed using the FlowJo TM Software (10.6.1). Cell sorting Cell populations were isolated using fluorescent-activated cell sorting (FACS) using the Beckman Coulter MoFlo Astrios with GFP laser (excitation wavelength 488 nm). Initial FSC/SCC was set between 30/40 and 210/240 to exclude debris. After removal of dead cells with Draq7 dye and removal of doublets, following standard protocol, cells were gated for sorting as can be seen in Fig. S1A . As a control, a non-GFP expressing tissue (forelimbs isolated from the same E12.5 embryos) was used to determine the gating of the GFP− fraction of the samples to sort. When multiple cell sortings were needed, gating was done in accordance to previous samples to ensure non-variability in GFP intensity. Flow cytometry analysis to obtain GFP histograms was performed with the FlowJo TM Software (version 10.6.1). Cell processing for ChIP-seq and Capture-HiC After sorting, cells were centrifuged for 5′ at 400 × g at 4 °C and supernatant was discarded. Cells for ChIP-seq and Capture-HiC were resuspended in 10% FCS/PBS and fixed in 1% formaldehyde for ChIP and 2% for Capture-HiC at room temperature. The fixation was blocked by the addition of 1.25 M glycine, cells were isolated by centrifugation (1000 × g , at 4 °C for 8’), resuspended in cold lysis buffer (10 mM Tris, pH 7.5, 10 mM NaCl, 5 mM MgCl 2 , 0.1 mM EGTA, Protease Inhibitor (Roche, 04693159001)) and incubated on ice for 10’ to isolate the cell nuclei. The nuclei were isolated by centrifugation (1000 × g , at 4 °C for 3′), washed in cold 1× PBS, centrifuged again (1000 × g , at 4 °C for 1’) and stored frozen at −80 °C after removal of the PBS supernatant. RNA-seq Cell processing and library preparation After sorting, cells were centrifuged for 5′ at 400 × g at 4 °C, supernatant was discarded and cells frozen at −80 °C. At least two biological replicates of 1.5 × 10 5 cells each were used to extract total RNA using the RNeasy Micro Kit (QIAGEN, ID:74004) following manufacturer’s instructions and then stored frozen at −80 °C. Total RNA was quantified with a Qubit (fluorimeter from Life Technologies) and RNA integrity assessed with a Bioanalyzer (Agilent Technologies). The SMART-Seq v4 kit from Clontech was used for the reverse transcription and cDNA amplification according to the manufacturer’s specifications, starting with 5 ng of total RNA as input. 200 pg of cDNA were used for library preparation using the Nextera XT kit from Illumina. Library molarity and quality was assessed with the Qubit and Tapestation using a DNA High sensitivity chip (Agilent Technologies). Libraries were pooled at 2 nM and loaded for clustering on a Single-read Illumina Flow cell for an average of 35 mio reads/library. Reads of 50 bases were generated using the TruSeq SBS chemistry on an Illumina HiSeq 4000 sequencer. ChIP-seq and library preparation 5 × 10 5 fixed nuclei were sonicated to a 200–500 bp length with the Bioruptor Pico sonicator (Diagenode). H3K27Ac ChIP (Diagenode C15410174) was performed as previously described [48] , [49] , using 1/500 dilution of the antibody, with the addition of 5 mM of Na-Butyrate to all buffers. Libraries were then prepared following the Illumina ChIP TruSeq protocol and sequenced as 50 bp single-end reads on a illumina HiSeq 4000. Libraries were prepared starting with below <10 ng quantities of ChIP-enriched DNA as starting material and processed with the Illumina TruSeq ChIP kit according to manufacturer specifications. Libraries were validated on a Tapestation 2200 (Agilent) and a Qubit fluorimeter (Invitrogen – Thermofisher Scientific). Libraries were pooled at 2 nM and loaded for clustering on a Single-read Illumina Flow cell. Reads of 50 bases were generated using the TruSeq SBS chemistry on an Illumina HiSeq 4000 sequencer. Capture-HiC and library preparation 3C libraries were prepared as previously described [48] . Briefly, at least 1 × 10 6 fixed cells were digested using the DpnII restriction enzyme (NEB, R0543M). Chromatin was re-ligated with T4 ligase (Thermo Fisher Scientific), de-crosslinked and precipitated. To check the validity of the experiment, 500 ng of re-ligated DNA were loaded on a 1% gel along with undigested and digested controls. 3C libraries were sheared and adapters ligated to the libraries according to the manufacturer’s instructions for Illumina sequencing (Agilent). Pre-amplified libraries were hybridized to the custom-designed SureSelect beads (chr13: 54,000,001–57,300,000) [11] ) and indexed for sequencing (50–100 bp paired-end) following the manufacturer’s instructions (Agilent). Enriched libraries were pooled at 2 nM and loaded for clustering on a Paired-End Illumina Flow cell for an average of 215 mio reads/library. Reads of 100 bases were generated using the TruSeq SBS chemistry on an Illumina HiSeq 4000 sequencer. ChIP-seq, RNA-seq and Capture-HiC  data analyses ChIP-seq Single-end reads were mapped to the reference genome NCBI37/mm9 using Bowtie2 version 2.3.4.2 [50] , filtered for mapping quality q ≥ 25 and duplicates were removed with SAMtools 1.9. Reads were extended to 250 bp and scaled (1 million/total of unique reads) to produce coverage tracks using genomecov of BEDTools/2.28.0-fecbf4e3. BigWig files were produced using bedGraphToBigWig version 4 and visualized in the UCSC genome browser. RNA-seq Single-end reads were mapped to the mm9 reference genome using STAR mapper version 2.5.2a with default settings. Further processing was done according to ref. [48] . BigWig files were visualized in the UCSC genome browser. Counting was done using R version 3.6.2 and differential expression was analyzed through the “DEseq2” R package (version 3.14). The DEseq2 R package was also used to produce heatmaps by subtracting from each gene value per condition, given by vst, the mean value of all conditions. Genes were picked according to adjusted p-value, all being significantly differentially expressed between conditions. Pitx1 fold enrichment between wildtype GFP+ and GFP− and between GFP−, GFP+− and GFP++ populations was calculated using Deseq2’s normalization by size factor with the addition of a 0.5 pseudocount to aid data visualization. The Wald-test was used to examine the differential across samples. The p -values were adjusted for multiple testing with the FDR/Benjamin–Hochberg (BH) method and each analysis was performed with at least two biological replicates. Expression heatmaps were generated for non-mesenchyme satellite and mesenchymal markers as defined in Supplementary Dataset S1 . For visualization reasons, Ccr5 , Cldn5, and Col2a1 were added as sub-cluster markers (endothelium immune and condensation) and the forelimb-specific marker Tbx5 was removed from the marker list. Moreover, genes with expression less or equal to 1 RPKM in all 8 samples (GFP+ wildtype: replicate 1 and 2; GFP− wildtype: replicate 1 and 2, GFP+ mutant: replicate 1 and 2; GFP− mutant: replicate 1 and 2) were removed from the analysis. For the GFP− specific heatmap, we additionally removed all genes with less or equal to 1 RPKM in all 4 GFP− samples. The color of the expression heatmap corresponds to the z-score transformed RPKM values, using the mean and standard deviation per gene based on all 8 samples. Log2FC was calculated by averaging replicates RPKM for each datasets and dividing Pitx1 GFP and Pitx1 GFP;ΔPen values. Capture-HiC and virtual 4C Paired-end reads from sequencing were mapped to the reference genome NCBI37/mm9 using with Bowtie2 version 2.3.4.2 [50] and further filtered and deduplicated using HiCUP version 0.6.1. When replicates were available, these were pooled through catenation (-cat in Python 2.7.11) before HiCUP analysis. Valid and unique di-tags were filtered and further processed with Juicer tools version 1.9.9 to produce binned contact maps from valid read pairs with MAPQ ≥ 30 and maps were normalized using Knights and Ruiz matrix balancing, considering only the genomic region chr13: 54,000,001–57,300,000 [51] , [52] , [53] . After KR normalization, maps were exported at 5 kb resolution. Subtraction maps were produced from the KR normalized maps and scaled together across their subdiagonals. C-HiC maps were visualized as heatmaps, where contacts above the 99thpercentile were truncated for visualization purposes. Further details about data processing can be accessed at ref. [11] . Virtual 4C profiles were generated from the filtered hicup.bam files used also for Capture-HiC analysis. The viewpoint for the Pitx1 promoter was set at coordinates chr13:55,930,001–55,940,000 (10 kb bin) and contact analysis was performed over the entire genomic region considered for Capture-HiC (chr13: 54,000,001–57,300,000). A contact pair is considered when one interaction fragment is in the viewpoint and its pair mate is outside of it. The interaction profile was smoothed by averaging over 5 kb intervals and was produced as a bedgraph file. Single-cell data analyses Processing of sequenced reads Demultiplexing, alignment, filtering barcode, and UMI counting was performed with 10× Genomics Cell Ranger software (version 3.0.2) following manufacture’s recommendations, default settings and mm10 reference genome (version 3.0.0, provided by 10X Genomics, downloaded in 2019). Cell Ranger outputs files for each dataset were processed using the velocyto run10x shortcut from velocyto.py tool [24] (version 0.17.17) to generate a loom file for each sample, using as reference genome the one provided by 10× Genomics and the UCSC genome browser repeat masker.gtf file, to mask expressed repetitive elements. Each loom matrix, containing spliced/unspliced/ambiguous reads, was individually imported in R (version 3.6.2) with the Read Velocity function from the Seurat Wrappers package (version 0.2.0). In parallel, feature filtered output matrices obtained from Cell Ranger were individually loaded into R through the Read10X function of the Seurat package (version 3.2.0 [54] ). Then, we combined the spliced, unspliced, ambiguous, and RNA feature data in a single matrix for each dataset. Subsequently each matrix was transformed into a Seurat object using Seurat package. Therefore, for each sample we obtained for each sample a single Seurat object comprehend by four assays, three of them (spliced, unspliced and ambiguous) were used for downstream RNA velocities estimations and the RNA feature assay was used for downstream gene expression analysis between the samples, as described below. Quality control and filtering Quality control and pre-processing of each Seurat object of our eight samples was performed attending to the following criteria. Cells expressing less than 200 genes were excluded. Additionally, we calculated the reads that mapped to the mitochondrial genome and we filtered out the cells with a mitochondrial content higher than 15%, since high levels of mitochondrial mRNA has been associated to death cells. Also, we excluded cells with a mitochondrial content lower than 1%, since we observed that these belong, in our datasets, to blood cells probably coming from the dissection protocol. Individual dataset normalization, scaling, and dimensional reduction After filtering, one by one we normalized the eight datasets following the default Seurat parameters for the LogNormalize method and applying it only to the RNA features assay. We next scaled it by applying a linear transformation and we calculated the most variable features individually for downstream analysis, using standard Seurat parameters. Scaled data were then used for principal component analysis (PCA), we used the 50 PCs established by default, and non-linear dimensional reduction by Uniform Manifold Approximation Projection (UMAP [55] ), we used 1:50 dims as input. Cell doublet identification Pre-process and normalized datasets were individually screened for detection of putative doublet cells. Doublets in each dataset were also excluded using DoubletFinder R package (version 2.0.2) [56] as described in https://github.com/chris-mcginnis-ucsf/DoubletFinder . The doublet rate (nExp parameter) used was estimated from the number of cells captured and it is as follows: Pitx1 +/+ Hindlimb replicate 1, nExp = 106; Pitx1 +/+ Hindlimb replicate 2, nExp = 123; Pitx1 +/+ Forelimb replicate 1, nExp = 97; Pitx1 +/+ Forelimb replicate 2, nExp = 116; Pitx1 − / − Hindlimb replicate 1, nExp = 104; Pitx1 − / − Hindlimb replicate 2, nExp = 122; Pitx1 Pen−/Pen− Hindlimb replicate 1, nExp = 118; Pitx1 Pen−/Pen− Hindlimb replicate 2, nExp = 116. The pK parameter was calculated following the strategy defined by ref. [56] and is as follow: Pitx1 +/+ Hindlimb replicate 1, pK = 0.12; Pitx1 +/+ Hindlimb replicate 2, pK = 0.005; Pitx1 +/+ Forelimb replicate 1, pK = 0.09; Pitx1 +/+ Forelimb replicate 2, pK = 0.04; Pitx1 − / − Hindlimb replicate 1, pK = 0.04; Pitx1 − / − Hindlimb replicate 2, pK = 0.01; Pitx1 Pen−/Pen− Hindlimb replicate 1, pK = 0.005; Pitx1 Pen−/Pen− Hindlimb replicate 2, pK = 0.005. After filtering, we kept for downstream analysis the following number of cells for each dataset: Pitx1 +/+ Hindlimb replicate 1, 4143 cells; Pitx1 +/+ Hindlimb replicate 2, 4816 cells; Pitx1 +/+ Forelimb replicate 1, 3802 cells; Pitx1 +/+ Forelimb replicate 2, 4521 cells; Pitx1 − / − Hindlimb replicate 1, 4049 cells; Pitx1 − / − Hindlimb replicate 2, 4745cells; Pitx1 Pen−/Pen− Hindlimb replicate 1, 4600 cells; Pitx1 Pen−/Pen− Hindlimb replicate 2, 4518 cells. Merge of all datasets and normalization Once each dataset was individually filtered and doublets were removed, all datasets were merged in a unique Seurat object without performing integration to execute an ensemble downstream analysis of the eight datasets. No batch effect was observed later on in this merged dataset. A new column to the Seurat object metadata was added to label replicates of the same tissue and animal model with the same name for downstream analysis. Therefore the cells of Pitx1 +/+ Hindlimb, replicate 1, and replicate 2 were labeled as Pitx1 +/+ Hindlimb, the same logic was applied to the rest of the samples. Subsequently, we normalized our new and unique Seurat object applying the SCTransform normalization protocol [57] , with default parameters, over the spliced assay. Cell-cycle scoring and regression Since from the individual analysis of our dataset we observed a part of the variance was explained by cell-cycle genes, we examine cell-cycle variation in the merged dataset. To do so we assigned to each cell a score based on its expression of a pre-determined list of cell cycle gene markers, following the strategy defined by [58] and by applying CellCycleScoring function implemented in Seurat. Subsequently, the evaluation of this results, we decided to regress out the cell-cycle heterogeneity. Therefore, we applied to our merged object the SCTransform normalization method, using the spliced assay as source, and adding to the default settings the cell-cycle calculated scores (S.Score and G2M.Scores) as variables to regressed. Cell Cycle classification was later on used to estimate cell cycle proportions on each cluster. Clustering After cell-cycle regression, cells were clustered using standard steps of the SCTransform Seurat workflow. Briefly, PCA (npcs = 50), UMAP (dims = 1:50) and nearest neighbors of each cell were calculated. Clusters were determined using Seurat FindClusters function with default parameters and a resolution of 0.2, in that way 10 clusters were defined. Identification of clusters identity was done by calculating the expression difference of each gene between each cluster and the rest of the clusters using the FindConservedMarkers function. We applied this function to each cluster (ident.1) using default parameters, only.pos = TRUE and setting as grouping variable the limb identity of the datasets, in that way we obtained a list of markers for each cluster independent of the limb sample. Clusters with similar marker were combined, therefore we finally worked with 5 clusters (Fig. 1B ): the mesenchyme (that contains 5 out of the 10 clusters), the epithelium (formed by 2 out of 10), and the immune cell cluster, the muscle and the endothelium clusters (composed by only 1 cluster each). We confirmed the expected identity markers were present in the new clustering by running the FindMarkers function with the following parameters logfc.threshold = 0.7; pseudocount.use = 0; only.pos = TRUE; min.diff.pct = 0.15 and all other default parameters (Supplementary Dataset S1 ). Subsetting and re-clustering Since the interest of this work was focus on the populations that in a wildtype hindlimb express Pitx1 (Fig. 1C ), we subsetted the mesenchyme cluster. To have a better insight on the different cell-types that integrate it, we re-cluster the mesenchyme cluster. To do so, UMAP embedding was calculated with the following parameters: dims = c(1:10), n.neighbors = 15L, min.dist = 0.01, metric = “cosine”, spread = 0.5, all other parameters were default. Cluster resolution after finding neighbors was established at 0.4 to reveal subpopulations. We observed 9 mesenchyme subpopulations (Fig. 3A ) that we named according to their identity genes. Identity markers were found using FindMarkers on the RNA assay, setting logfc.threshold = 0.3, pseudocount = 0, min.diff.pct = 0.1, only.pos = TRUE and all other parameters as default (Supplementary Dataset S1 ). Differential expression analysis To perform Pitx1 +/+ Hindlimb vs Pitx1 Pen−/Pen− Hindlimb differential expression analysis in the mesenchyme cluster and in each one of the nine mesenchyme clusters we used the FindMarkers function on the RNA assay. For whole mesenchyme analysis Pitx1 Pen−/Pen− Hindlimb was set up as ident.1 and Pitx1 +/+ Hindlimb as ident.2. To determine the differentially expressed genes between each dataset in each mesenchyme cluster, we created a new column in the metadata slot that contains both cluster and dataset information. Then, this column was set as new identity and differential expression analysis was run using as ident.1: ICT_Pitx1 Pen − /Pen − , Ms_Pitx1 Pen − /Pen − , TP_Pitx1 Pen − /Pen − , LDC_Pitx1 Pen − /Pen − , DPP_Pitx1 Pen − /Pen − , DP_Pitx1 Pen − /Pen − , PC_Pitx1 Pen − /Pen − , EDC_Pitx1 Pen − /Pen − , or PPP_Pitx1 Pen − /Pen − and as ident.2: ICT_HL_Pitx1 +/+ , Ms_HL_Pitx1 +/+ , TP_HL_Pitx1 +/+ , LDC_HL_Pitx1 +/+ , DPP_HL_Pitx1 +/+ , DP_HL_Pitx1 +/+ , PC_HL_Pitx1 +/+ , EDC_HL_Pitx1 +/+ or PPP_HL_Pitx1 +/+ . All the other parameters as default except setting logfc.threshold = 0.2, pseudocount.use = 0 (Supplementary Dataset S5 ). RNA-velocity analysis As input data for the RNA-velocity analysis, we used the unspliced (pre-mature) and spliced (mature) abundances calculated for each replicate of our datasets as explained above (see in Methods, Processing of sequencing reads). To perform the RNA velocity analysis on the mesenchyme clusters of each dataset we subset the cells belonging to the 2 replicates. Therefore, we subset Pitx1 +/+ Hindlimb, Pitx1 +/+ Forelimb, Pitx1 Pen − /Pen − Hindlimb, and Pitx1 − / − Hindlimb individually. We also performed RNA-velocity analysis of all combined datasets. To perform proximal clusters and distal clusters analysis, we subset them separately following the criteria for proximal and distal cluster classification that is explained below in the Methods. Seurat objects from which we performed RNA-velocity analysis were saved as h5Seurat file using SeuratDisk package (version 0.0.0.9013) and exported to be used as input of Scvelo (version 0.2.2) [59] in Python (version 3.7.3). Then the standard protocol described in scVelo was followed. Standard parameters were used except npcs = 10 and n.neighbors = 15, to be the same that we used for the UMAP embedding in Seurat. Differential proportion analysis Statistical differential proportion analysis, to study the differences in clusters cell proportions between the different limb-type conditions, was performed in R using the source code published by [60] after generating the proportion tables in R. Null distribution was calculated using n = 100,000 and p = 0.1 as in the original reference. Pairwise comparisons were performed between the different condition tested. Proximal and distal cell classification Proximal, distal or NR attribute was given to each cluster based on its Shox2 and Hoxd13 expression. 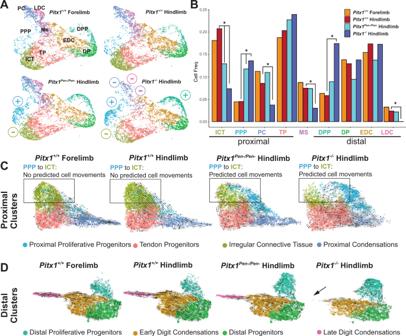Fig. 5: Influence of thePendeletion on limb cell populations. AUMAP of mesenchymal cell type proportions across conditions, (+) and (−) symbols indicate increase or decrease in cell proportions in comparison to wildtype hindlimbs. Abbreviations are described in Fig.2A.BQuantification of cell type proportions across conditions,p-values < 0.01 are marked with an asterisk (see Source data).P-values were calculated pairwise using differential proportion analysis in R60. Abbreviations are described in Fig.2A.CVelocity analyses from proximal clusters in all dataset. Arrows represent the direction toward the predicted fate territories. Note inPitx1Pen−/Pen−andPitx1−/−the velocity-predicted cell movements between PPP and ICT which likely represent ongoing differentiation that is not predicted in wildtype hindlimbs or forelimbs.DVelocity analyses from distal clusters in all dataset. Note inPitx1−/−hindlimbs the loss of late digit condensations (black arrows) at the end of the velocity-predicted cell movements. Therefore, ICT, TP, PPP, and PC clusters were classified as proximal clusters, DP, DPP, EDC, and LDC as distal ones. Meanwhile Ms cluster that express both markers were not classify to any of them. This classification was added to the Seurat object metadata and used in downstream analysis. Pitx1 density plot and cell classification by Pitx1 expression Pitx1 normalized expression values (using Seurat default LogNormalize method, using log1p), from the RNA assay of the all dataset merged Seurat Object, were extracted in a data frame. This data frame was used to create a density plot using ggplot2 package (version 3.3.2). From the overlay of Pitx1 density distributions in the Pitx1 +/+ Hindlimb and the Pitx1 Pen − /Pen − Hindlimb samples we define the intersection point of 0.3 to classify cells in non/low-expressing and expressing cells. 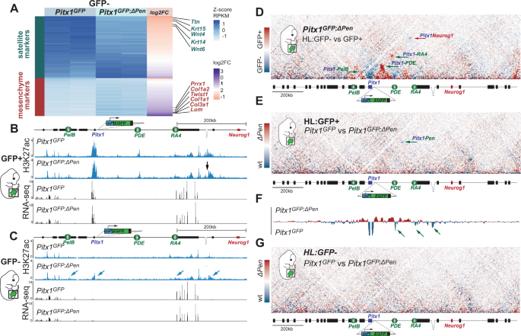Fig. 6: Single enhancer deletion results in inefficient regulatory landscape activation. ALog2 fold change and RPKM of mesenchymal (red) and satellite (darkgreen) marker genes inPitx1GFPandPitx1GFP;ΔPenGFP− hindlimbs cells. Note the decrease in satellite markers and the increase in mesenchymal markers inPitx1GFP;ΔPenGFP− cells.BH3K27ac ChIP-seq and RNA-seq tracks at thePitx1locus in GFP+ cells ofPitx1GFPandPitx1GFP;ΔPenhindlimbs. Note the loss of thePenenhancer region (black arrow).CH3K27ac ChIP-seq and RNA-seq at thePitx1locus in GFP− cells ofPitx1GFPandPitx1GFP;ΔPenhindlimbs. Note the acetylation ofPitx1promoter and enhancers (blue arrows) and the weakPitx1transcription.DC-HiC subtraction map between GFP− and GFP+Pitx1GFP;ΔPenhindlimb cells. GFP+ preferential interactions are displayed in red and GFP- preferential interactions in blue.EC-HiC subtraction maps betweenPitx1GFPandPitx1GFP;ΔPenGFP+ hindlimb cells. Note the loss of interaction betweenPitx1and thePen-deleted region (green arrow).Pitx1GFP;ΔPenGFP+ preferential interactions are displayed in red andPitx1GFPGFP+ preferential interactions in blue.FSubtraction track of virtual 4C betweenPitx1GFP(blue) andPitx1GFP;ΔPen(red) GFP+ hindlimb cells with thePitx1promoter as viewpoint. Note the partial loss of interactions betweenPitx1and its telomeric enhancers (PDE, RA4, andPen; green arrows).GC-HiC subtraction maps betweenPitx1GFPandPitx1GFP;ΔPenGFP− hindlimb cells.Pitx1GFP;ΔPenGFP− preferential interactions are displayed in red andPitx1GFPGFP− preferential interactions in blue. 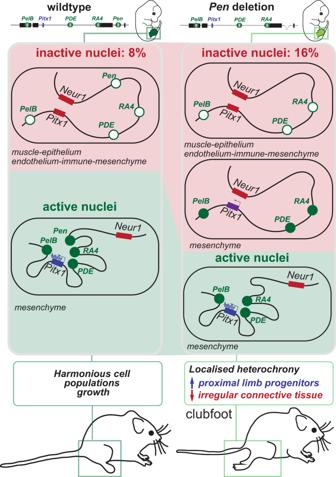Fig. 7: Model. In wildtype hindlimb tissues (left panel) 8% of the nuclei, mostly from non-mesenchymal origin, display a completely repressedPitx1locus, featured by inactive enhancers (white ovals), polycomb-repressedPitx1gene (red rectangle) and inactive 3D chromatin structure (Pitx1does not contact its enhancers but contacts the repressedNeurog1gene). In active nuclei, the situation is inverted with active enhancers (green ovals), active 3D chromatin structure (Pitx1contacts its enhancers) and strongPitx1transcription. In contrast, in hindlimb lacking thePenenhancer (right panel), 16% of the cells are lackingPitx1transcription. Among these cells, some display a partially active regulatory landscape. These latter cells, that have failed to establish an active 3D structure and a strongPitx1transcription, are of mesenchymal origins in particular of ICT and PPP types. The remaining active cells in mutant hindlimbs appear to display wildtype expression levels. Phenotypically, the effect of the enhancer deletion is a disharmonious outgrowth of cell populations featured by a gain of PPP and a decrease of ICT cells. This cellular phenotype is likely at the origin of the clubfoot phenotype. The second intersection point of 1.45 that subclassify these expressing cells in intermediate- and high- expressing cells was established based on the intersection of the Pitx1 +/+ Hindlimb proximal and distal cells (Fig. 2F ). Therefore, we classified as non/low- expressing cells those with Pitx1 expression values <0.3, as intermediate-expressing those with Pitx1 expressing values between >0.3, <1.45 and as high-expressing cells those >1.45. This classification and Pitx1 expression values were added as new columns to the Seurat object metadata and used in downstream analysis. Reporting summary Further information on research design is available in the Nature Research Reporting Summary linked to this article.